Contrasting role of antimony and bismuth dopants on the thermoelectric performance of lead selenide Increasing the conversion efficiency of thermoelectric materials is a key scientific driver behind a worldwide effort to enable heat to electricity power generation at competitive cost. Here we report an increased performance for antimony-doped lead selenide with a thermoelectric figure of merit of ~1.5 at 800 K. This is in sharp contrast to bismuth doped lead selenide, which reaches a figure of merit of <1. Substituting antimony or bismuth for lead achieves maximum power factors between ~23–27 μW cm −1 K −2 at temperatures above 400 K. The addition of small amounts (~0.25 mol%) of antimony generates extensive nanoscale precipitates, whereas comparable amounts of bismuth results in very few or no precipitates. The antimony-rich precipitates are endotaxial in lead selenide, and appear remarkably effective in reducing the lattice thermal conductivity. The corresponding bismuth-containing samples exhibit smaller reduction in lattice thermal conductivity. Advances in high-performance thermoelectric materials can potentially impact electrical power generation through waste-heat recovery [1] , [2] , [3] . Such thermoelectric materials demand high value of the dimensionless figure of merit (ZT) defined as ZT =( S 2 σ /κ) T ( T is the temperature, S is the Seebeck coefficient, σ is the electrical conductivity, and κ is the total thermal conductivity (comprising κ el and κ lat ; representing contributions from charge carriers and lattice, respectively) for practical applications. Combining ZT and Carnot efficiency determines the efficiency of thermoelectric energy conversion. Thus, increasing such conversion efficiency requires both high ZT and a large temperature gradient across the materials. One effective way to achieve high ZT is to reduce lattice thermal conductivity through embedding micro/nanostructures, which provide multiple scattering mechanisms for phonons [1] , [2] , [4] , [5] , [6] , [7] , [8] , [9] , [10] , [11] , [12] , [13] , [14] , [15] , [16] , [17] , [18] . Other strategies address the challenge of maximizing a power factor from existing semiconducting materials by band alignment [5] , [6] , [19] , [20] , modifying their electronic structures close to the Fermi level [21] , [22] , and increasing band degeneracy by convergence of bands [23] . The rocksalt-structured lead chalcogenide semiconductors have many compelling attributes as promising thermoelectric materials. As one of the most investigated materials in this system, lead telluride (PbTe) has been extensively studied. PbTe remains the top-performing thermoelectric at mid-temperature range (600–900 K). However, concerns regarding the scarcity of tellurium (Te) in the Earth’s crust [24] are motivating the development of materials based on more abundant elements. Lead selenide (PbSe), a much lower cost analogue of PbTe, is an attractive alternative as selenium (Se) has a better long-term price stability and lower cost than Te; and is ~50 times more abundant than Te [24] . Moreover, PbSe has much higher melting temperature (1,357 K) than PbTe (1,198 K) that may enable a higher efficiency for the same value of ZT at higher operating temperatures. Recently, high ZT values have been reported for n-type PbSe ( ZT =~0.9 for PbSe-In/Ga (ingot) [25] and ~1.2 (hot-pressed samples) [26] at 900 K, ~0.8 at 700 K for PbSe-Cl [27] , ~1.2 at 850 K for PbSe-Br [28] , ~1.3 at 850 K for PbSe-Al [29] and ~1.3 at 900 K for PbSe/PbS-Cl [9] ). Advances also have been reported for p-type PbSe ( ZT =~1.2 at 850 K for PbSe-Na [30] , ~1.0 at 770 K for PbSe-Ag [31] , ~1.0 at 700 K for PbSe-Tl [26] , ~1.3 at 900 K for PbSe/(Sr/Ba)Se-Na [4] and ~1.6 at 900 K for PbSe/CdS-Na [5] ). Theoretical calculations have suggested that heavily doped p-type PbSe can potentially show a ZT ~2 at 1,000 K [32] and n-type PbSe can be a high-performance thermoelectric as well because of large thermopower [33] , which offers added motivation for investigations in this system. Here, we report contrasting high-temperature thermoelectric properties of PbSe doped with antimony (Sb) and bismuth (Bi). Sb and Bi act as n-type dopants and enable tuning of the carrier concentration by substituting nominal Sb 3+ /Bi 3+ for Pb 2+ in the rock-salt sublattice. We demonstrate that Sb not only has merely the simple role as a dopant for carrier generation but that, unexpectedly, it is also remarkably effective in generating a unique form of nanostructuring that dramatically reduces the lattice thermal conductivity of PbSe. The surprising fact is that even very small amounts (≤0.25 mol%) of Sb in PbSe generate a highly dense array of well dispersed nanostructures. In sharp contrast to Sb, Bi dopant generates only few nanoscale precipitates, if any, and does not notably affect the lattice thermal conductivity of PbSe. We have employed the pulsed electric current sintering technique, also known as spark plasma sintering, to obtain highly dense and robust thermoelectric specimens starting from mesoscale powders. We report high ZT values that peak at different temperatures based on Sb concentration. We observe a ZT of ~1.2 at 700 K for Pb 0.99875 Sb 0.00125 Se, ~1.5 at 830 K for Pb 0.9975 Sb 0.0025 Se, ~1.4 at 930 K for Pb 0.995 Sb 0.005 Se and ~1.2 at 930 K for samples of Pb 0.9925 Sb 0.0075 Se and Pb 0.99 Sb 0.01 Se; which represent highest reported ZT values for such systems. In contrast, all respective Bi-containing PbSe samples exhibit ZT <1. As explained below, the contrasting behaviour of Sb- and Bi-doped PbSe lies in the remarkably different microstructure evolution, primarily in the nanoscale. 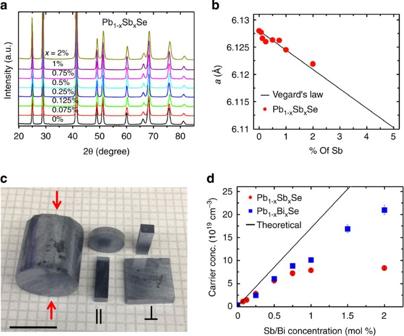Figure 1:PXRD and Hall charge-carrier concentration of Pb1−xSbxSe and Pb1−xBixSe. (a) PXRD patterns for samples of Pb1−xSbxSe. (b) lattice parameters as a function of Sb concentration. (c) Typical spark plasma sintering pellet and samples used in this study. Red arrows indicate the pressing direction. Results of parallel to the pressing direction measurements are shown in the text and perpendicular direction measurements are in the supporting information. Scale bar, 1 cm. (d) Hall-effect charge-carrier concentration in Pb1−xSbxSe and Pb1−xBixSe samples. The solid line is the predicted carrier concentration. Structural characterization Figure 1a presents the Powder X-ray diffraction (PXRD) patterns of Pb 1− x Sb x Se samples. All patterns were indexed in the NaCl structure ( Fm -3 m space group) without any noticeable second phase (within the detection limit of our X-ray diffraction equipment) for Sb contents of up to 2 mol%. Figure 1b shows the extracted lattice parameters as a function of Sb content. The lattice parameter of PbSe decreases with increasing Sb content. This is Vegard’s law behaviour, and it is consistent with size trends (Sb is smaller than Pb) and indicates some solubility of the Sb ions in the lattice. As we will show, however, the key feature of this system is the extensive nanostructuring created in the PbSe matrix that is detectable with only with transmission electron microscopy (TEM). Figure 1c shows a typical spark plasma sintering disk-shaped pallet cut and polished for measurements in this study. Both directions (parallel and perpendicular to pressing direction) were measured and showed no directional dependence. Only results of parallel direction measurements are shown in the text and perpendicular direction measurements are in the Supplementary Fig. 1 . Figure 1: PXRD and Hall charge-carrier concentration of Pb 1− x Sb x Se and Pb 1− x Bi x Se. ( a ) PXRD patterns for samples of Pb 1− x Sb x Se. ( b ) lattice parameters as a function of Sb concentration. ( c ) Typical spark plasma sintering pellet and samples used in this study. Red arrows indicate the pressing direction. Results of parallel to the pressing direction measurements are shown in the text and perpendicular direction measurements are in the supporting information. Scale bar, 1 cm. ( d ) Hall-effect charge-carrier concentration in Pb 1− x Sb x Se and Pb 1− x Bi x Se samples. The solid line is the predicted carrier concentration. Full size image Charge-carrier concentration and electron mobility In this study, Sb and Bi were used as dopants and from simple valence counting each atom is expected to add one extra n-type carrier to PbSe. In Fig. 1d , the room temperature Hall carrier-concentrations are plotted as a function of the added amount of dopant. Table 1 also shows a summary of the physical properties of the samples. Here, the solid line represents one electron per Sb/Bi atom added. For both Sb and Bi samples, the experimental values fall well below the theoretical ones. In particular, for Sb samples from 0.75 mol%, the values of experimental Hall charge-carrier concentration almost reach saturation, while Bi samples exhibit almost linearly increasing carrier concentration. This suggests that Bi is significantly more soluble in PbSe than Sb and the Hall measurements indicate that the carrier saturation of Sb is reached at ~0.75 mol% Sb, and that of Bi is not reached even up to 2 mol% Bi. The lower than expected carrier concentration values of Sb-containing samples are attributed to nanostructuring as explained below. Table 1 Thermoelectric properties of Pb 1− x (Sb/Bi) x Se samples. Full size table The electrical conductivity ( σ ) of Pb 1− x Sb x Se samples is depicted in Fig. 2a (corresponding results of Pb 1− x Bi x Se samples are shown in Fig. 3a ). For all samples, a monotonic decrease in σ with increasing temperature is observed, consistent with heavily doped semiconductors with metallic transport behaviour. For Sb-containing samples, the electrical conductivity increases with increase in Hall carrier concentration at any given temperature. However, the electrical conductivity at lower temperature decreases for 1.5 mol% and 2 mol% of Bi-containing samples despite the higher Hall carrier concentrations. This can be explained by the possibility of increasing impurity scattering from the higher doping (See Supplementary Note 1 ). 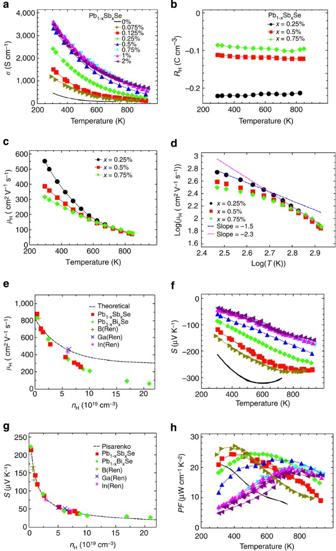Figure 2:Electrical transport properties of Pb1−xSbxSe. (a)Temperature dependence of electrical conductivity of Pb1−xSbxSe. (b) Hall coefficient as a function of temperature forx=0.25, 0.5 and 0.75% containing Pb1−xSbxSe samples. Note that the Hall coefficient is almost temperature independent. (c) Hall mobility as a function of temperature forx=0.25, 0.5, and 0.75% containing Pb1−xSbxSe samples. (d) log(μH)–log(T) plot showing two regions of linearity, one below 475 K and the other above 500 K. The high-temperature region is characterized by a much steeper slope reflecting a strong electronic-scattering mechanism at play. (e) Room temperature Hall mobility for Pb1−xSbxSe and Pb1−xBixSe samples as a function of the experimental Hall charge-carrier concentration. (f) Temperature-dependent Seebeck coefficient of Pb1−xSbxSe samples. (g) Room temperature Seebeck coefficient for Pb1−xSbxSe and Pb1−xBixSe samples as a function of the experimental Hall charge-carrier concentration. (h)Temperature-dependent thermoelectric power factor of Pb1−xSbxSe samples. Data for PbSe doped with B, Ga, In by Zhanget al.26Black dashed line is due to the model described in the text. Figure 2: Electrical transport properties of Pb 1− x Sb x Se. ( a )Temperature dependence of electrical conductivity of Pb 1− x Sb x Se. ( b ) Hall coefficient as a function of temperature for x =0.25, 0.5 and 0.75% containing Pb 1− x Sb x Se samples. Note that the Hall coefficient is almost temperature independent. ( c ) Hall mobility as a function of temperature for x =0.25, 0.5, and 0.75% containing Pb 1− x Sb x Se samples. ( d ) log( μ H )–log( T ) plot showing two regions of linearity, one below 475 K and the other above 500 K. The high-temperature region is characterized by a much steeper slope reflecting a strong electronic-scattering mechanism at play. ( e ) Room temperature Hall mobility for Pb 1− x Sb x Se and Pb 1− x Bi x Se samples as a function of the experimental Hall charge-carrier concentration. ( f ) Temperature-dependent Seebeck coefficient of Pb 1− x Sb x Se samples. ( g ) Room temperature Seebeck coefficient for Pb 1− x Sb x Se and Pb 1− x Bi x Se samples as a function of the experimental Hall charge-carrier concentration. ( h )Temperature-dependent thermoelectric power factor of Pb 1− x Sb x Se samples. Data for PbSe doped with B, Ga, In by Zhang et al. [26] Black dashed line is due to the model described in the text. 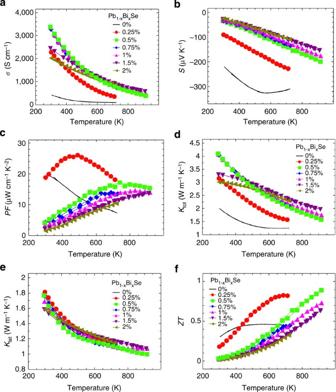Figure 3:Thermoelectric properties of Pb1−xBixSe. (a) Temperature-dependent electrical conductivity, (b) Seebeck coefficient, (c) thermoelectric power factor, (d) total thermal conductivity, (e) lattice thermal conductivity and (f) thermoelectric figure of merit of Pb1−xBixSe samples. Full size image Figure 3: Thermoelectric properties of Pb 1− x Bi x Se. ( a ) Temperature-dependent electrical conductivity, ( b ) Seebeck coefficient, ( c ) thermoelectric power factor, ( d ) total thermal conductivity, ( e ) lattice thermal conductivity and ( f ) thermoelectric figure of merit of Pb 1− x Bi x Se samples. Full size image To understand the behaviour of σ , we performed temperature-dependent Hall-effect studies. The Hall coefficient, R H , for the Sb-containing samples for x =0.25, 0.5, and 0.75% is plotted in Fig. 2b which shows it is almost temperature independent. Hall-effect measurements can determine the carrier densities under the assumption of a unitary of single band transport and a Hall coefficient R H =1/ n H e , where n H is the Hall charge-carrier density and e is the electron charge. The temperature-independent Hall coefficient shows that the specimens retain the same carrier density up to 850 K. Figure 2c presents the Hall mobility, μ H = R H σ , as a function of temperature. The room temperature μ H values decrease from~550 cm 2 V −1 s −1 for 0.25% of Sb to~310 cm 2 V −1 s −1 for 0.75% of Sb, because of enhanced point defect scattering with increasing doping level. At high temperature, a rapid decrease is observed and μ H =~70 cm 2 V −1 s −1 at 850 K for all three samples. The rapid decrease of μ H is shown more clearly on a log( μ H )-log( T ) plot in Fig. 2d . In the temperature range from 300 K to 475 K, the slopes of the curves are ~−1.2, but for T>500 K the slopes increase to ~−2.4. Table 2 summarizes the fitting results. This type of mobility exponent is characteristic of scattering mechanisms that are related to the band structure parameters. Assuming parabolic bands, electron–phonon scattering due to thermal vibrations of the lattice cause μ H to scale as μ H ~T −1.5 (ref. 34 ). The low-temperature exponent in Fig. 2d can be attributed to acoustic phonon scattering of electrons in agreement with previous results on highly doped PbSe samples [35] . In both the work of Gobrecht and Schlichting [36] and our data, the exponent changes and approaches −1 as concentrations increase, again in good agreement with theory and experimental data for the effective mass. At high-temperature, strong electronic-scattering mechanisms, non-parabolicity of the bands and/or scattering from high-frequency vibrations of the lattice (optical phonons) possibly have a role to rapidly decrease the values of exponents at high temperature [37] , [38] . Table 2 Characteristic slopes of the log( μ H )-log( T ) for Pb 0.9975 Sb 0.0025 Se, Pb 0.995 Sb 0.005 Se and Pb 0.9925 Sb 0.0075 Se samples for two different temperature regimes. Full size table The experimental transport data were analysed with solutions to the Boltzmann transport equations within the relaxation time approximation. It is assumed that electron conduction occurs within a single parabolic band considering multiple ellipsoidal valleys with degeneracy N c=4, where in the same valley the effective masses along different directions of the ellipsoids are different. The different effective masses give rise to band anisotropy, which is defined as K = m l */ m t * where m l * is the effective mass associated with the longitudinal axes of the ellipsoidal energy surfaces, and m t * associated with two of the transverse axis of the surfaces. In the case of PbSe, the band anisotropy factor is K =1.75 [39] , [40] . The equations shown below are valid for a single-scattering mechanism where the energy dependence of the carrier relaxation time can be expressed by a simple power law. Thus, the relaxation time, τ, has a simple power law dependence on the charge-carrier energy, ε, so τ( T ,ε)=τ 0 ( T )ε λ− 1/2 , here τ 0 is the energy-independent term of the relaxation time, and λ is the scattering parameter. For acoustic phonon scattering λ=0, and it will be assumed that this is the dominant scattering mechanism. Note that some representations may differ by the factor of −1/2 (ref. 41) [41] . Within the approximations outlined above, the Hall mobility can be expressed as [42] : Here, is the conductivity-effective mass defined as . The Fermi integrals F n ( η ) are the Fermi integrals defined by May et al. [43] and evaluated for a specific reduced chemical potential, η =E F /kT . The energy-independent term of the relaxation time in the case of acoustical phonon scattering is defined [28] Here, C l =9.1 × 10 10 Pa is a combination of elastic constants [44] , [45] , and E def is the deformation potential, which describes the carrier-scattering strength by acoustic phonons. Ravich et al. [39] listed a room temperature deformation potential of 20 eV, while Wang et al. [28] gave a value of 25 eV for n-type PbSe. The effective mass in the denominator of equation (2) defined as is the mass of a single valley, which is related to the total density of states mass via [40] For a specific η , the Hall mobility as calculated by equation (1) can be related to the Hall charge-carrier concentration through: where the Hall factor, r H , is defined by [43] In Fig. 2e , the room temperature Hall mobility values of n-type PbSe samples as well as data reported by Ren and coworkers [26] are plotted as a function of Hall charge-carrier concentration. From equation (2), τ 0 = 8.9 × 10 −14 s was obtained and a temperature constant E def =29 eV, close to the literature values mentioned above [39] , and a density of states effective mass of m *=0.36 m e , where m e is the free electron mass were used, in agreement with the effective mass obtained from the carrier dependence of the Seebeck coefficient discussed in the succeeding section. As seen from Fig. 2e , the theoretical line describes well the experimental data up to carrier densities ~3 × 10 19 cm −3 , but highly Sb/Bi-containing samples fall below the values expected by the model. We have to notice that the same fitting quality was found assuming single spherical surfaces [43] ; however, the obtained effective mass was found underestimated relative to the one obtained from the Pisarenko plot discussed below. The disagreement between the calculated and the experimental room temperature mobility of Fig. 2e may be attributed to non-parabolicity of bands, microscopic cracks, grain boundaries and defects leading to a higher residual resistance, and consequently, a lower Hall mobility. As it is shown in the Supplementary Fig. 2 and Supplementary Note 2 , the conduction band non-parabolicity was found to be the major deterrent effect for the description of the carrier dependence of Hall mobility within the framework of a single parabolic model. However, the Seebeck coefficient was found to be well described by the simple parabolic band model in the whole composition range and this is the model we have used to calculate the reduced chemical potentials and the Lorenz numbers. Seebeck coefficient and power factor Figure 2f shows the Seebeck coefficients ( S ) of Pb 1− x Sb x Se samples as functions of temperature (corresponding results of Pb 1− x Bi x Se samples are shown in Fig. 3b ). As expected, the S values are negative over the entire temperature range, indicating n-type conduction. Most samples show almost degenerate linear behaviour. The magnitudes (absolute values) of the S of the low Sb-containing samples display maxima at high temperature, where thermally activated holes reduce the thermoelectric voltage. In Fig. 2g , the absolute Seebeck coefficients for n-type PbSe samples are plotted as a function of the Hall charge-carrier concentration (Pisarenko plot) at room temperature. Data from this study and the literature [26] are compared with a theoretical calculation. The dashed black curve is calculated using a single parabolic model. In this model, dominated by acoustic phonon scattering outlined above, the Seebeck coefficient is given by [42] : The S can be related to n H through equation (4) provided the effective mass, m *, is known. The dashed line shown in Fig. 2g is generated by assuming a same effective mass of m *=0.36 m e that is used in the calculation of theoretical mobility and agrees well with the experimental data for all n-type PbSe. Figure 2h presents power factors derived from the electrical conductivities and Seebeck coefficients as a function of temperature for Pb 1− x Sb x Se samples (corresponding results of Pb 1− x Bi x Se samples are in Fig. 3c ). As expected, the maximum for the power factor is pushed to higher temperatures as the amount of dopant is increased. Whereas the x =0% sample have its maxima at ~300 K, the x =0.075 and 0.125% samples have their maximum at ~400 K, the x =0.25% sample at ~500 K, the x =0.5% sample at ~650 K, and the x ≥0.75% at ~800 K and all the maximum values are large enough (≥19 μW cm −1 K −2 ) for good thermoelectric properties. This shows that varying the dopant concentration controls the temperature of optimum thermoelectric performance. Thermal conductivity The temperature dependence of total thermal conductivity is shown in Fig. 4a (corresponding results of Pb 1− x Bi x Se samples are shown in Fig. 3d ). The total thermal conductivity (κ tot ), which consists of contributions from the charge carriers (κ el ) and the lattice phonons (κ lat ), decreases with decreasing Hall charge-carrier concentration and increasing temperature. The charge-carrier thermal conductivity is directly proportional to the electrical conductivity that derives from the Wiedmann–Franz relation κ el = LσT , where L is the Lorenz number. 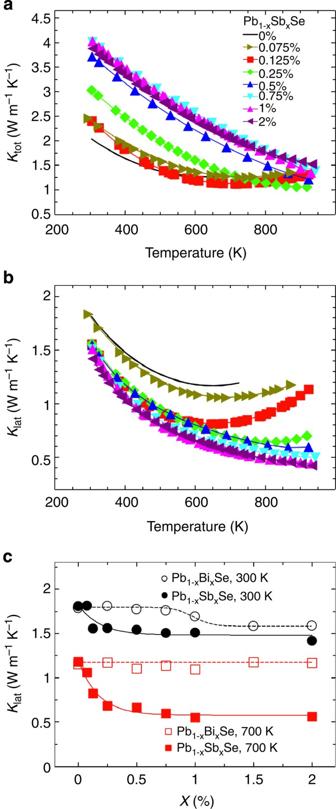Figure 4:Thermal transport properties of Pb1−xSbxSe. (a) Temperature dependence of total thermal conductivity and (b) lattice thermal conductivity of Pb1−xSbxSe samples. (c) Lattice thermal conductivity of Pb1−xSbxSe samples (filled) and Pb1−xBixSe samples (empty) shown as a function of x at 300 K (black) and 700 K (red). Solid and dashed lines are guide to the eye. In the assumption of a homogeneous material with a parabolic band dominated by acoustic phonon scattering, the Lorenz number is given as [42] , [46] : Figure 4: Thermal transport properties of Pb 1− x Sb x Se. ( a ) Temperature dependence of total thermal conductivity and ( b ) lattice thermal conductivity of Pb 1− x Sb x Se samples. ( c ) Lattice thermal conductivity of Pb 1− x Sb x Se samples (filled) and Pb 1− x Bi x Se samples (empty) shown as a function of x at 300 K (black) and 700 K (red). Solid and dashed lines are guide to the eye. Full size image The reduced chemical potential was obtained from fits of the experimental Seebeck coefficient. Using these chemical potential values, L and κ el for each sample can be calculated and are shown in Supplementary Figs 3 and 4 . The lattice thermal conductivities (κ lat ) for Pb 1− x Sb x Se samples are shown in Fig. 4b (corresponding results of Pb 1− x Bi x Se samples are shown in Fig. 3e ). The lattice thermal conductivity decreases with increasing temperature for x ≥0.5% of Sb samples but lower doping samples show upturn at high temperature (more details in the Supplementary Fig. 3 ). The x =0.075% sample shows similar κ lat values to that of pristine sample. However, for x ≥0.125% samples, κ lat decreases compared to pristine samples. The room temperature κ lat decrease from ~1.81 Wm −1 K −1 for both pristine PbSe and x =0.075% to ~1.56 W m −1 K −1 , ~1.56 W m −1 K −1 , ~1.54 W m −1 K −1 , ~1.51 W m −1 K −1 , ~1.51 W m −1 K −1 and 1.42 W m −1 K −1 for x =0.125, 0.25, 0.5, 0.75, 1 and 2% of Sb, respectively (See Table 1 and Fig. 4c ). The reduction of κ lat is even greater at higher temperature. At 700 K, κ lat decrease from ~1.18 W m −1 K −1 , ~1.06 W m −1 K −1 , ~0.82 W m −1 K −1 , ~0.68 W m −1 K −1 , ~0.66 W m −1 K −1 , ~0.60 W m −1 K −1 , ~0.55 W m −1 K −1 and ~0.56 W m −1 K −1 for x =0, 0.075, 0.125, 0.25, 0.5, 0.75, 1 and 2% of Sb, respectively (See Table 1 and Fig. 4c ). The lowest value of ~0.42 W m −1 K −1 is obtained at 930 K for x =2% sample. Clearly, very large reductions in the Sb system are observed. In contrast, Pb 1− x Bi x Se shows no such effects and instead similar κ lat values to that of pristine PbSe are observed. The room temperature κ lat is ~1.79 W m −1 K −1 , ~1.81 W m −1 K −1 , ~1.77 W m −1 K −1 , ~1.76 W m −1 K −1 , ~1.69 W m −1 K −1 , ~1.58 W m −1 K −1 and ~1.59 W m −1 K −1 for x =0, 0.25, 0.5, 0.75, 1, 1.5 and 2% of Bi, respectively (See Table 1 and Fig. 4c ). By adding Bi to PbSe matrix, the high temperature κ lat does not change either. The κ lat at 700 K is ~1.15 W m −1 K −1 , ~1.17 W m −1 K −1 , ~1.10 W m −1 K −1 , ~1.13 W m −1 K −1 , ~1.10 W m −1 K −1 , ~1.17 W m −1 K −1 and ~1.16 W m −1 K −1 for for x =0, 0.25, 0.5, 0.75, 1, 1.5 and 2% of Bi, respectively (See Table 1 and Fig. 4c ). Even the lowest value of Bi system is quite high with ~1.00 W m −1 K −1 at 920 K for x =0.5%. Nanostructuring and TEM The very large reductions in lattice thermal conductivity of the Sb-containing system can be explained by understanding the microstructure, particularly at the nanoscale. Typical low- and medium-magnification bright field TEM images of Pb 1− x Sb x Se samples are shown in Fig. 5 . The low-magnification TEM images of 0.5% Sb-doped sample, acquired respectively along [001] ( Fig. 5a ) and [011] zone axes ( Fig. 5b ), show the dark-strain contrast from the precipitates. In the corresponding selected-area electron diffraction (SAED) patterns (insets in Fig. 5a,b ), which include both the matrix and the precipitates, only Bragg spots consistent with that of PbSe can be observed, confirming crystallographic alignment (endotaxy) of the nanoscale precipitates and matrix. Shown in Fig. 5c–f are the atomic-scale high-resolution TEM images. When the electron beam is parallel to the [001] zone axis ( Fig. 5c,e,f ), the precipitates appear as dark straight and thick line-segments with length of a few nanometres that are orthogonal to each other in about equal proportion. The directions normal to these projected lines are either [010] or [100] as indicated. When the beam is oriented along [011] zone axis ( Fig. 5d ), most of the precipitates appear to have quasi-circular (oval) and elongated shape. These observations are consistent with an oval disc-shaped morphology of Sb-rich precipitates with three crystallographic variants, along three sets of {100} planes. 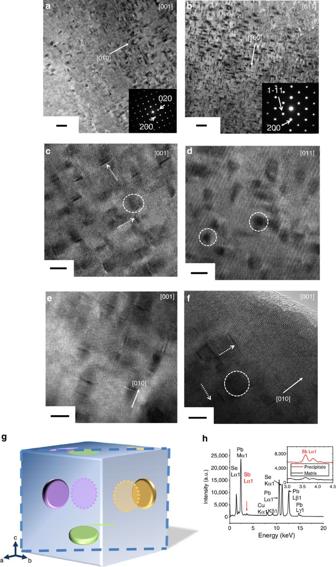Figure 5:TEM and EDS spectra of Pb1−xSbxSe. (a) Low-magnification TEM images of Pb0.995Sb0.005Se along the [001] and (b) [011] zone axes. The insets show the SAED patterns. (c) Medium-magnification TEM images of Pb0.995Sb0.005Se along the [001] and (d) [011] zone axes, (e) Pb0.9975Sb0.0025Se, and (f) Pb0.99925Sb0.00075Se, both along the [001] zone axis. The arrows and circle shown in (c) indicate the oval disc and elongated shapes of the precipitates. (g) schematic illustration of the three crystallographic variants of oval disc-shape precipitates. (h), EDS spectra of Pb0.9Sb0.1Se sample from the precipitate The inset is the magnified Sb peak comparing between the precipitate and the matrix. Scale bar, 20 nm (a,b), 5 nm (c–f). Figure 5c shows two such obvious variants orthogonal to each other, while the third variant is within the thin foil with normal to the field of view; which is expected to have low contrast, as indicated by the dotted arrows and the circle, respectively. Figure 5d confirms the elongated sectional view expected for [011] matrix orientation. Figure 5g shows the schematic illustration of the three variants of the oval disc-shaped precipitates parallel to {100}, and with their projection along ‹001› and ‹011› directions. Figure 5: TEM and EDS spectra of Pb 1− x Sb x Se. ( a ) Low-magnification TEM images of Pb 0.995 Sb 0.005 Se along the [001] and ( b ) [011] zone axes. The insets show the SAED patterns. ( c ) Medium-magnification TEM images of Pb 0.995 Sb 0.005 Se along the [001] and ( d ) [011] zone axes, ( e ) Pb 0.9975 Sb 0.0025 Se, and ( f ) Pb 0.99925 Sb 0.00075 Se, both along the [001] zone axis. The arrows and circle shown in ( c ) indicate the oval disc and elongated shapes of the precipitates. ( g ) schematic illustration of the three crystallographic variants of oval disc-shape precipitates. ( h ), EDS spectra of Pb 0.9 Sb 0.1 Se sample from the precipitate The inset is the magnified Sb peak comparing between the precipitate and the matrix. Scale bar, 20 nm ( a , b ), 5 nm ( c – f ). Full size image The number density of these oval disc-shaped precipitates increases with increasing Sb fraction. A high number of well-defined nanoscale precipitates is observed for the Pb 0.995 Sb 0.005 Se samples. High-number density of precipitates is also observed for samples with x≥0.125% of Sb ( Fig. 5e ) that exhibit considerably reduced κ lat . These characteristics point to additional scattering mechanisms arising from the matrix-nanoscale precipitate interfaces, mass-contrast effects as well as accompanying spatially varying strain. In contrast, the even more dilute Pb 0.99925 Sb 0.00075 Se sample ( Fig. 5f ) showed few or no precipitates and its κ lat is similar to that of the pristine compound, strongly suggesting that nanostructure scattering mechanism for heat-carrying phonons is not prevalent for much diluted Sb-doped samples. The existence of Sb in the nanoscale precipitates was confirmed by energy dispersive spectroscopy (EDS; Fig. 5h ) for Pb 0.9 Sb 0.1 Se samples, which contain similar nanoscale precipitates and morphology; and are conducive to EDS analysis given larger amount of Sb in these samples. The main EDS spectrum shown in Fig. 5h was obtained when the beam was focused at a precipitate. As shown in the inset of Fig. 5h , the relative intensity of the Sb Lα1 peak is higher when the beam is focused at the precipitates (red line) compared with the matrix (black line). Unlike Sb-doped samples, Bi-doped samples do not exhibit nanostructures ( Supplementary Fig. 5 ), suggesting that it forms solid solution with matrix PbSe, and thereby explains why Bi-doped samples show similar κ lat as pristine PbSe. One of the primary goals of this investigation was to determine the evolution of κ lat with changing dopants (Sb versus Bi) and their amount (mol% fraction). In Fig. 4c , the lattice thermal conductivity at 300 K and 700 K is plotted as a function of x for both Pb 1− x Sb x Se and Pb 1− x Bi x Se. In the Pb 1− x Sb x Se samples, there is a marked decrease in κ lat with the addition of even fewer per cent of Sb at both 300 and 700 K. The decrease in κ lat is more dramatic at high temperature. The values of κ lat at 300 K and 700 K for Pb 1− x Bi x Se samples are shown for comparison. Adding Bi seems to slightly reduce κ lat values at room temperature but there is almost no effect at high temperature. Thus, all κ lat values at 700 K for Bi samples up to x =2% are similar to the value of pristine PbSe. This trend suggests that the solubility limit of Sb is ~0.125 mol% Sb, but that of Bi is ≥2 mol% Bi. In addition to the lack of nanoscale precipitates, the lower mass contrast between Pb and Bi further reduces the prospects for additional phonon scattering mechanism. In Fig. 6a , the Hall mobility at 300 K is presented as a function of x for both Pb 1− x Sb x Se and Pb 1− x Bi x Se. The Sb-rich endotaxial nanocrystals in the PbSe matrix do not appear to affect the electron scattering. Pb 1− x Sb x Se samples have even better mobility than Pb − x Bi x Se samples that lack nanostructuring. A possible reason for this is the endotaxy of Sb-rich precipitates in PbSe that leaves fewer point defects of Sb dissolved in the Pb sublattice. By comparison, the more soluble Bi creates more point defects directly in the Pb sublattice and raises the probability of electron scattering. This confluence of endotaxially arranged Sb-rich nanocrystals effectively inhibiting heat flow in the system, but not electron flow, allows for the large power factor to be achieved. 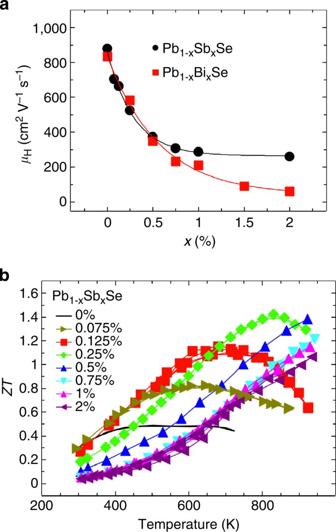Figure 6:Contrast between Pb1−xSbxSe and Pb1−xBixSe andZTof Pb1−xSbxSe. (a) Mobility of Pb1−xSbxSe samples (black) and Pb1−xBixSe samples (red) shown as a function of x at room temperature. Solid lines are guide to the eye. (b), the thermoelectric figure of merit as a function of temperature for Pb1−xSbxSe samples. Figure 6: Contrast between Pb 1− x Sb x Se and Pb 1− x Bi x Se and ZT of Pb 1− x Sb x Se. ( a ) Mobility of Pb 1− x Sb x Se samples (black) and Pb 1− x Bi x Se samples (red) shown as a function of x at room temperature. Solid lines are guide to the eye. ( b ), the thermoelectric figure of merit as a function of temperature for Pb 1− x Sb x Se samples. Full size image Thermoelectric figure of merit Figure 6b depicts the temperature dependence of ZT for Pb 1− x Sb x Se samples (corresponding results of Pb 1− x Bi x Se samples are shown in Fig. 3f ). Combining high-power factors and low-thermal conductivity gives high ZT values. The highest ZT of ~1.5 at 830 K is observed for the Pb 0.9975 Sb 0.0025 Se sample. This system outperforms other bulk n-type PbSe systems and might be able to control the different optimal temperatures with varying dopant concentration. This value matches the best n-type PbTe-based materials. We find high ZT values over the large temperature range as the content of Sb is tuned. Thus, ZT values of ~0.8 at 600 K for Pb 0.99925 Sb 0.00075 Se, ~1.2 at 700 K for Pb 0.99875 Sb 0.00125 Se, ~1.5 at 830 K for Pb 0.9975 Sb 0.0025 Se, ~1.4 at 930 K for Pb 0.995 Sb 0.005 Se, and ~1.2 at 930 K for Pb 0.9925 Sb 0.0075 Se and Pb 0.99 Sb 0.01 Se samples are observed. In comparison, ZT values for all Bi samples are lower than 1 (~0.83 at 690 K for Pb 0.99925 Bi 0.00075 Se, ~0.89 at 920 K for Pb 0.995 Bi 0.005 Se, ~0.73 at 920 K for Pb 0.99 Bi 0.01 Se and ~0.63 at 910 K for Pb 0.985 Bi 0.015 Se). Counter to expectations, Sb in PbSe does not behave as an ideal dopant. A very small amount of Sb causes a surprisingly extensive nanostructuring in PbSe, resulting in dramatic increase in thermoelectric performance. It is remarkable that only 0.25 mol% of Sb can generate such an extensive array of well-defined endotaxial nanoscale precipitates that do not reduce power factor and function predominantly as strong phonon scatterers, particularly at high temperature. As a result, ZT of ~1.5 is achieved for this system at 830 K, the highest ever reported for PbSe-based systems. This essentially matches the highest ZT value of any n-type PbTe-based materials. The addition of Bi instead seems to lead to ideal dopant behaviour, that is, solid solution formation and carrier generation but has no other beneficial effect on thermal conductivity reduction compared with pristine PbSe. From this work, it is apparent that PbSe-based materials are now emerging as promising, less expensive alternatives to PbTe that have the potential for enabling energy conversion devices with good thermoelectric performance at higher operating temperatures, exceeding the traditional PbTe-based materials. The results reported here for n-type PbSe samples coupled with the previous achievement of high ZT ~1.6 in p-type PbSe samples, propel the PbSe system to the higher echelons of the group of top-performing thermoelectric materials composed of more earth abundant elements. We believe these results open new vistas for broad-based viable high-temperature thermoelectric power generation applications and high-temperature waste-heat utilization. Synthesis Ingots (~20 g ) with nominal compositions Pb 1− x Sb x Se ( x =0, 0.00075, 0.00125, 0.0025, 0.005, 0.0075, 0.01 and 0.02) and Pb 1− x Bi x Se ( x =0.0025, 0.005, 0.0075, 0.01, 0.015 and 0.02) were prepared by mixing appropriate ratios of reagents in quartz tubes. The tubes were sealed under vacuum (~10 −4 Torr) and heated up to 1,150 °C over a period of 12 h, soaked at that temperature for 5 h and rapidly cooled to room temperature over 3 h. The obtained ingots were cleaned and ground to a powder using a mechanical grinder to reduce the particle sizes to <53 μm. These powders were densified at 650 °C for 5 min under an axial compressive pressure of 40 MPa in an argon atmosphere. The relative densities were achieved in the range of 97.8–100% of theoretical values (see Supplementary Information). PXRD PXRD patterns for all samples were collected using Cu Kα radiation on an INEL diffractometer operating at 40 kV and 20 mA equipped with a position sensitive detector. Electrical properties The samples for charge transport properties measurement were cut and polished into a parallelepiped with dimensions of ~2 mm × 3 mm × 10 mm. The electrical conductivity and Seebeck coefficient were measured simultaneously under a helium atmosphere (~0.1 atm) from room temperature to ~923 K using an ULVAC-RIKO ZEM-3 system. Samples measured to 923 K were coated with boron nitride to protect the instrument and the sample against evaporation of elements. Multiple cycles and different specimens produced similar properties. Hall measurement The charge transport specimens were subsequently used in room temperatures Hall-effect measurements to determine their carrier densities on the assumption of a unitary Hall factor, which gives a Hall coefficient, R H =1/ n H e , where n H is the Hall charge-carrier density and e is the electronic charge. Hall coefficients were measured in a home-built system in a magnetic field ranging from 0.5 to 1.25 T, utilizing a simple four-contact Hall-bar geometry, in both negative and positive polarity of the magnetic field to eliminate Joule-resistive errors. The high-temperature Hall coefficient was measured for selected Sb-containing samples ( x =0.25, 0.5, 0.75%) in a homemade high-temperature apparatus under argon atmosphere, which provides a working range from 300 to 850 K. The charge transport specimens polished to thin slab samples with dimensions of ~1 mm × 2 mm × 8 mm were used. The Hall resistance was recorded with a Linear Research ac resistance bridge (model LR-700), which was operated at 17 Hz. The magnetic field was provided by an air-bore Oxford superconducting magnet and the data were taken from 0.5 to −0.5 T. The carrier concentration is calculated from the same assumption of a unitary Hall factor. The values of carrier concentration at room temperature are similar to those from room temperature Hall-effect measurement within 5% error. The mobility values, μ , at room temperature were calculated from the relation μ H = σ/n H e . Thermal conductivity A NETZSCH LFA 457 MicroFlash instrument was used to determine the thermal diffusivity of samples cut and polished to rectangular parallelepipeds for perpendicular direction measurement and disk-shape for parallel direction measurement ( Fig. 1c ) coated with graphite. Thermal conductivity is calculated from κ= DC p d , where D is the thermal diffusivity, C p is the heat capacity, and d is the density. The specific heat per unit mass of the PbSe was used literature values [47] of the heat capacity of PbSe: Supplementary Fig. 6 shows the heat capacities obtained in the thermal diffusivity measurement using a pyroceram 9606 standard. The literature heat capacity is in good agreement with these data. The mass-density values used here were calculated using the geometrical dimensions of the specimens measured with a digital caliper and mass measured on a four-digit balance; corresponding densities were ≥97.8% theoretical density. The details of D and d are shown in Supplementary Fig. 7 , and Supplementary Table 1 . TEM The samples were characterized under the JEOL 2100F S/TEM operated at 200 kV. Thin TEM specimens were prepared by conventional methods and include cutting, grinding, dimpling, polishing and low-energy Ar-ion milling equipped with a liquid nitrogen cooling stage. How to cite this article: Lee, Y. et al. Contrasting role of antimony and bismuth dopants on the thermoelectric performance of lead selenide. Nat. Commun. 5:3640 doi: 10.1038/ncomms4640 (2014).